Molecular basis of transmembrane beta-barrel formation of staphylococcal pore-forming toxins Pathogenic bacteria secrete pore-forming toxins (PFTs) to attack target cells. PFTs are expressed as water-soluble monomeric proteins, which oligomerize into nonlytic prepore intermediates on the target cell membrane before forming membrane-spanning pores. Despite a wealth of biochemical data, the lack of high-resolution prepore structural information has hampered understanding of the β-barrel formation process. Here, we report crystal structures of staphylococcal γ-haemolysin and leucocidin prepores. The structures reveal a disordered bottom half of the β-barrel corresponding to the transmembrane region, and a rigid upper extramembrane half. Spectroscopic analysis of fluorescently labelled mutants confirmed that the prepore is distinct from the pore within the transmembrane region. Mutational analysis also indicates a pivotal role for the glycine residue located at the lipid–solvent interface as a ‘joint’ between the two halves of the β-barrel. These observations suggest a two-step transmembrane β-barrel pore formation mechanism in which the upper extramembrane and bottom transmembrane regions are formed independently. Pathogenic bacteria secrete various virulence factors to attack host cells. Pore-forming toxins (PFTs) are among the most sophisticated virulence factors. PFTs are expressed as water-soluble monomeric proteins, which assemble on the membranes of the target cells to form membrane-inserted pores [1] . With the appearance of the pore on the membrane, the cells are killed through leakage. It is interesting to note that PFTs are expressed not only by pathogenic bacteria but also by eukaryotic cells as immune proteins, such as perforin and complement C9. This suggests that PFTs are universally used in a wide range of organisms [2] . PFTs can be classified into two families according to the secondary structure of the transmembrane region, that is, α-helical PFTs and β-barrel PFTs (β-PFTs) [3] , [4] . Staphylococcus aureus , a major cause of hospital- and community-acquired infections, secretes several β-PFTs, including α-haemolysin (α-HL), γ-haemolysin (γ-HL), leucocidin (LUK) and Panton–Valentine leucocidin, to kill blood cells [5] . α-HL consists of a single polypeptide, whereas the others require two different components, that is, class F and class S-components. γ-HL, LUK and Panton–Valentine leucocidin are composed of LukF and Hlg2, LukF and LukS, and LukF-Panton–Valentine (PV) and LukS-PV, as class F- and S-components, respectively. The components of bicomponent β-PFTs have amino-acid sequence similarity to each other: within a class, proteins are ~70% identical, while the level of identity drops to ~30% between classes. Class F proteins are more closely related to α-HL (~30%) than class S proteins (~20%) [5] , [6] . Previous biochemical experiments have suggested a general pore formation mechanism in which the soluble monomeric component assembles into a ring-shaped pore via a nonlytic oligomeric intermediate known as a prepore [7] , [8] . At the prepore stage, the β-barrel transmembrane pore has not yet formed, whereas a ring-shaped oligomer is formed [9] , [10] , [11] , [12] . The crystal structures of the monomeric form of α-HL [13] and several bicomponent PFTs, that is, LukF [14] , LukF-PV [15] , Hlg2 (ref. 16 ) and LukS-PV [17] , have been determined. In addition, crystal structures of the heptameric pore of α-HL [18] , [19] , [20] and octameric pore of γ-HL [21] have been determined. Four molecules of each of LukF and Hlg2 alternately assemble in a circular pattern in the γ-HL pore, whereas seven α-HL protomers assemble in a circular arrangement in the α-HL pore. These mushroom-shaped membrane pores commonly consist of three domains, that is, the cap, rim and stem domains. The cap domain is composed of β-sandwiches from each protomer. The rim domain consists of four β-strands with a loop-rich structure, and lies beneath the cap domain. The stem domain forms an antiparallel β-barrel, the bottom half of which comprises the transmembrane portion of the pore. The stem region is packed within the cap domain in the monomers, which is called the prestem. The prepore state octamer of the γ-HL structure model was constructed by superposing monomeric structures onto the pore [21] . In the prepore model, the prestems are packed inside the ring composed of the cap domains. Based on the crystal structures of the monomer and pore in combination with the prepore structure model, the following pore formation mechanism was proposed [21] . Each monomeric component assembles on the target cell membrane into a prepore with the prestem packed inside. After forming the prepore, a marked conformational change occurs on the packed prestem, and then the β-barrel pore is formed all at once. However, the proposed pore formation mechanism has a serious problem in that the prestem held inside has mutual steric hindrance. Thus, the structure of the actual prepore should differ from the model, and it is necessary to determine the actual structure of prepore to determine the pore formation mechanism. The prepore does not remain stable and proceeds immediately to pore formation once formed. However, mutation of two residues responsible for binding with the phospholipid head group located at the bottom of the rim domain of LukF, that is, Trp177 and Arg198, was reported to result in formation of a stable ring-shaped oligomer, although the transmembrane pore was not formed [10] . This means that the observed oligomer was in the state just before pore formation, that is, the prepore state. In the present study, we determined the crystal structures of the γ-HL oligomer using LukF W177A/R198A mutant (γ-HL-WR). In addition, the crystal structures of LUK were also determined. These analyses revealed the prepore structures of staphylococcal β-PFTs. It should be noted that staphylococcal PFT is the only family of which crystal structures of all members are available, which allows us to discuss the dynamics of the pore formation mechanism based on the actual structures of each stage. Based on the structural information and biochemical data, we propose a two-step transmembrane β-barrel pore formation mechanism. Crystal structure of γ-HL W177A/R198A mutant (γ-HL-WR) A previous study showed that LukF double mutant with Trp177 and Arg198 can exist stably as a prepore-like oligomer with Hlg2 (ref. 10 ). Therefore, the crystal structure of this mutant was expected to yield insight into the details of the β-barrel formation mechanism of staphylococcal β-PFTs. Moreover, we found previously that γ-HL (LukF and Hlg2) spontaneously formed pores in the presence of 2-methyl-2,4-pentanediol (MPD) [21] . In this study, we applied this technique to γ-HL-WR to determine the structure of the prepore. Crystals were grown in the presence of 60% MPD and the structure was determined at 2.99 Å. Although molecular replacement and cell content analysis showed that two molecules of the octamer were contained in an asymmetric unit, the electron density of one was too obscure to construct a structure model. In contrast, the other molecule had a clear electron density map. Therefore, we constructed and refined only one octamer molecule that had a clear electron density map. A similar disappearance of electron density for a large region was reported for gene product 12 of T4 bacteriophage [22] . No MPD molecules were bound around the lipid-head-binding site, in contrast to the structures of wild-type γ-HL and α-HL capturing MPD. Finally, R work / R free values converged to 23.0%/25.4%. As expected, the determined structure was an octamer in which four molecules of LukF and Hlg2 were alternately located in a circular pattern as reported previously for the γ-HL pore [21] ( Fig. 1a ). However, a critical difference was observed in that the bottom half of the β-barrel (Gly120–Gly135 of LukF and Gly114–Gly127 of Hlg2) was completely invisible, whereas the upper half showed clear electron density ( Fig. 1b ). The invisible region has a glycine-rich sequence in both LukF and Hlg2 (six and five Gly residues, respectively) ( Supplementary Fig. 1 ). Moreover, this region corresponds to residues located under an aromatic residue layer, which is commonly observed near the lipid/solvent interface of transmembrane β-barrels [23] , [24] . Other regions, that is, the upper half of the β-barrel, cap and rim domains, were successfully constructed with clear electron density. In addition, the N -terminal amino latch of Hlg2, which was disordered in the pore structure, was observed inside the cap domains. Compared with the wild-type pore, there were no significant differences in relative orientation among the upper half of the β-barrel, cap and rim domains ( Fig. 1c ). Therefore, the structure was superposed well onto that of the pore with r.m.s.d. of 0.22 Å for 1,920 Ca atoms ( Fig. 1c ). These observations indicated that only the transmembrane region of the β-barrel is disordered with no conformational change in other regions except the amino latch, which agreed with the molecular properties of γ-HL-WR with which it forms an oligomer with no haemolytic activity [10] . These structural characteristics strongly indicate that the upper and bottom halves of the β-barrel are formed independently. The observations that the first and end residues of the flexible region are Gly, and that the flexible transmembrane region is abundant in Gly residues suggest important roles of these Gly residues in the β-barrel pore formation process. 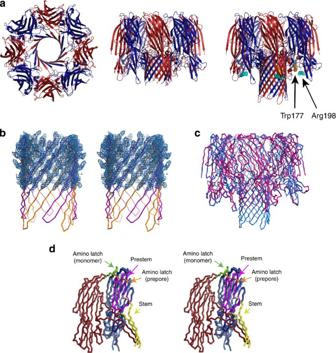Figure 1: Crystal structure of the γ-HL-WR prepore. (a) Overall structure, top view (left) and side view (centre). As a reference, the γ-HL pore is also shown in side view (right). LukF and Hlg2 are shown in red and blue, respectively. Arg198 and Trp177 are shown as orange and cyan ball models, respectively. The right figure was reproduced from (ref.21). (b) Stereo representation of 2Fo-Fc electron density map of the β-barrel contoured at 1.2 σ. Cα trace of the whole β-barrel is also shown. Orange: LukF, magenta: Hlg2. (c) Superposition of the octamer of γ-HL-WR (magenta) and wild-type pore reported previously (blue). (d) Stereo representation of Hlg2 protomer superposed on LukS-PV monomer (PDB 1T5R). Amino latch and prestem in monomer are shown in green and purple, respectively, and those of the prepore are shown in orange and yellow, respectively. To indicate the location of the adjacent protomer, LukF is also shown in red. Figure 1: Crystal structure of the γ-HL-WR prepore. ( a ) Overall structure, top view (left) and side view (centre). As a reference, the γ-HL pore is also shown in side view (right). LukF and Hlg2 are shown in red and blue, respectively. Arg198 and Trp177 are shown as orange and cyan ball models, respectively. The right figure was reproduced from (ref. 21 ). ( b ) Stereo representation of 2Fo-Fc electron density map of the β-barrel contoured at 1.2 σ. Cα trace of the whole β-barrel is also shown. Orange: LukF, magenta: Hlg2. ( c ) Superposition of the octamer of γ-HL-WR (magenta) and wild-type pore reported previously (blue). ( d ) Stereo representation of Hlg2 protomer superposed on LukS-PV monomer (PDB 1T5R). Amino latch and prestem in monomer are shown in green and purple, respectively, and those of the prepore are shown in orange and yellow, respectively. To indicate the location of the adjacent protomer, LukF is also shown in red. Full size image As described above, the present structure revealed the location of the N-terminus amino latch in oligomeric assembly. Figure 1d shows a structural comparison of the Hlg2 protomer in γ-HL-WR with monomeric LukS-PV. The amino latch in γ-HL-WR occupied a region in which the prestem was located in the monomer ( Fig. 1d ). In contrast, the amino latch in the monomer was located in the vicinity of the cap domain as a β-strand. In γ-HL-WR, this area was used for interacting with the adjacent protomer. These observations revealed a conformational change and a role of the amino latch in the pore formation process (see Discussion). Differences in the β-barrel between γ-HL and γ-HL-WR Crystal structure analysis showed that the difference between the pore and the prepore is whether the bottom half of the β-barrel is formed or not. To evaluate their structural differences on erythrocyte, six cysteine mutants of the β-barrel region were constructed for Hlg2 (V105C, L109C, I113C, S122C, S126C and S132C) and the fluorescence emission spectra of their derivatives in which fluorescent dye (6-bromoacetyl-2-dimethylaminonaphthalene (BADAN)) was conjugated via the introduced cysteine were measured. Ile113, Ser122 and Ser126 are located in the bottom half of the β-barrel, whereas others are located in the upper region ( Fig. 2a ). All of these BADAN-labelled Hlg2 mutants showed complete γ-HL activity to human erythrocytes with wild-type LukF, but no haemolysis was observed with LukF-WR. Before the spectroscopic measurement, each mutant was incubated with wild-type LukF or LukF-WR in the presence of erythrocyte membrane ghosts, which represent spectra for pore and prepore, respectively. 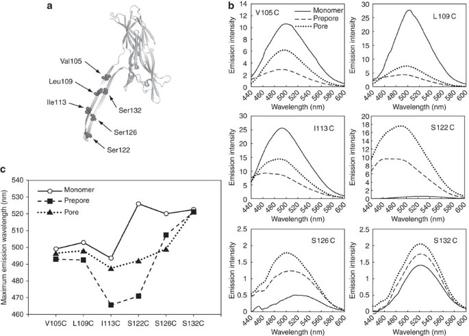Figure 2: Fluorescence-detected differences between prepore and pore. (a) Locations of the BADAN-labelled sites. (b) Fluorescence emission spectra of each mutant. Monomeric Hlg2 (solid line), prepore formed by incubation with LukF-WR mutant (dashed line) and pore prepared by incubation with LukF (dotted line) are shown. All spectra were corrected for background emission using the samples without BADAN-labelled protein. Each depicted net emission scan is the average obtained from three separate samples. (c) Peak wavelength of each spectrum (monomer: open circles, prepore: closed squares, pore: closed triangles). Figure 2b shows the spectral change of each mutant. The peak wavelength represents the microenvironment surrounding the conjugated BADAN, that is, blue and red shifts indicate burial into the hydrophobic environment and exposure to the hydrophilic environment, respectively. BADAN introduced in the bottom half, that is, I113C, S122C and S126C, induced a significant difference in shape of the spectrum between pore and prepore, which resulted in a difference in the peak wavelength ( Fig. 2b,c ). In contrast, other mutants had peaks at similar wavelengths in pore and prepore ( Fig. 2c ). These observations suggested that the environment around the bottom half of the β-barrel is different between the prepore and pore, whereas the upper region is similar, which was consistent with the results of crystal structure analysis indicating that the prepore had a similar structure as the pore but the transmembrane region is disordered. Figure 2: Fluorescence-detected differences between prepore and pore. ( a ) Locations of the BADAN-labelled sites. ( b ) Fluorescence emission spectra of each mutant. Monomeric Hlg2 (solid line), prepore formed by incubation with LukF-WR mutant (dashed line) and pore prepared by incubation with LukF (dotted line) are shown. All spectra were corrected for background emission using the samples without BADAN-labelled protein. Each depicted net emission scan is the average obtained from three separate samples. ( c ) Peak wavelength of each spectrum (monomer: open circles, prepore: closed squares, pore: closed triangles). Full size image Effects of substitution of Gly in the disordered region Crystal structure analysis suggested the importance of flexibility of the transmembrane region due to abundant Gly residues. To validate this suggestion, five mutants with substitution of Pro for Gly in the flexible transmembrane region were constructed for LukF (G120P, G121P, G131P, G132P and G135P) and their haemolytic activities towards rabbit erythrocytes were compared ( Fig. 3a ). All mutants except G135P showed decreased haemolytic activity, although the extent of inactivation was variable. Substitution of Gly120 caused complete loss of activity. G121P and G132P showed approximately half of the wild-type activity. Substitution of Gly131 decreased the activity by approximately 20%. Gly120, substitution of which caused complete inactivation, is the first residue of the region that was invisible on the electron density map, and is expected to be located at the lipid/solvent interface ( Supplementary Fig. 2A ). Other invisible residues were expected to be located in the transmembrane region. These observations indicated that flexibility conferred by Gly120 at the junction between the trans- and extramembrane regions plays a pivotal role in the haemolytic activity, although flexibility of the whole transmembrane region due to the abundant glycine residues is also important. 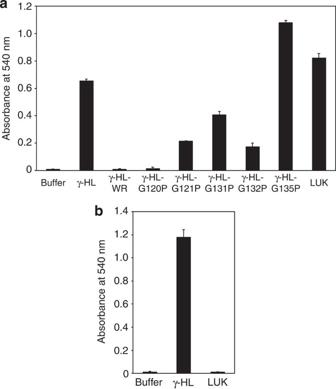Figure 3: Haemolytic activity of γ-HL mutants and LUK. Haemolytic activity of γ-HL mutants and LUK for rabbit erythrocytes (a) and human erythrocytes (b). The graphs show average values from three individual experiments and the corresponding s.d. Figure 3: Haemolytic activity of γ-HL mutants and LUK. Haemolytic activity of γ-HL mutants and LUK for rabbit erythrocytes ( a ) and human erythrocytes ( b ). The graphs show average values from three individual experiments and the corresponding s.d. Full size image In contrast to these inactivated mutants, G135P showed an increase in haemolytic activity by approximately 1.7-fold compared with the wild-type. Gly135 is located at the lipid/solvent interface of the β-strand returning to the rim domain ( Supplementary Fig. 2A ). This means that two Gly residues located at the lipid/solvent interface have opposite effects; that is, G120P inactivated the haemolytic activity, while G135P upregulated the activity. Gly120 and Gly135 are located in a β-strand going towards the top of the β-barrel and in that returning to the rim domain, respectively ( Supplementary Fig. 2A ). The dynamic role of the glycine residues located at the interface may differ according to whether the β-strand is going out or coming back. Application to other staphylococcal PFTs To confirm whether the pore formation mechanism proposed for γ-HL is commonly applicable to other PFTs and/or to verify that the observed structural properties are not caused by the mutations, the crystal structure of wild-type LUK in the presence of MPD was analysed. LUK is another staphylococcal two-component PFT, which is composed of LukF and LukS. Although LUK and γ-HL commonly utilize LukF as an F-component, they use different S-components, that is, γ-HL uses Hlg2, whereas LUK uses LukS. Due to the difference in the S-component, LUK and γ-HL show significant differences in target cell specificity [7] . γ-HL possesses activity for both rabbit and human erythrocytes, whereas LUK shows haemolytic activity only for rabbit erythrocytes ( Fig. 3 ). Despite the lack of activity towards human erythrocytes, electron microscopy revealed that LUK forms ring-shaped particles, which look like membrane pores of γ-HL in size on human erythrocytes ( Supplementary Fig. 3 ). These observations suggested that LUK forms stable prepores on human erythrocytes. The structure of wild-type LUK was determined at 2.4-Å resolution. The revealed structure showed structural characteristics that were quite similar to those of γ-HL-WR; that is, the transmembrane region was disordered, whereas other regions were well constructed ( Fig. 4 ). Sequence alignment showed that the invisible region of LUK was completely identical to that of γ-HL-WR ( Supplementary Fig. 1 ). As wild-type LUK, which shows full haemolytic activity towards rabbit erythrocytes, exhibited structural features identical to γ-HL-WR [25] , disorder of the transmembrane region was not an artefact of substitution of Trp177 and Arg198, but reflected the intrinsic nature of the molecule. It should be noted that a space for the transmembrane region was occupied by the rim domain of the adjacent octamer in the crystal ( Supplementary Fig. 4 ), suggesting that formation of the transmembrane region is not sterically allowed. Thus, the revealed structure should be definitely different from the pore. These observations strongly support the β-barrel pore formation mechanism proposed above for γ-HL-WR. In addition, MPD molecules were captured at the lipid-head-binding site of LukF as observed for the crystal structure of wild-type γ- and α-HL [20] , [21] ( Fig. 4c ). 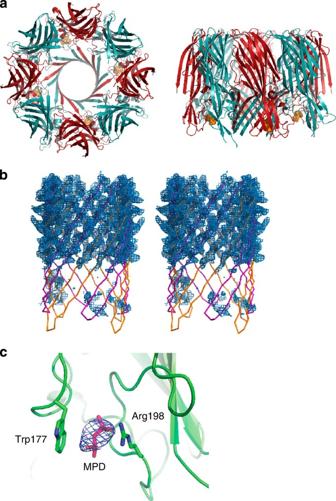Figure 4: Crystal structure of prepore of LUK. (a) Overall structure, top view (left) and side view (right). LukF and LukS are shown in red and cyan, respectively. (b) Stereo representation of 2Fo-Fc electron density map of the β-barrel contoured at 1.2 σ. Cα trace of the whole β-barrel structure of γ-HL is also shown. Orange: LukF, magenta: Hlg2. (c) Close-up view of the MPD-binding site. The bound MPD is shown as sticks. The Fo-Fc map (contoured at 1.5 σ) around the MPD is also shown. Figure 4: Crystal structure of prepore of LUK. ( a ) Overall structure, top view (left) and side view (right). LukF and LukS are shown in red and cyan, respectively. ( b ) Stereo representation of 2Fo-Fc electron density map of the β-barrel contoured at 1.2 σ. Cα trace of the whole β-barrel structure of γ-HL is also shown. Orange: LukF, magenta: Hlg2. ( c ) Close-up view of the MPD-binding site. The bound MPD is shown as sticks. The Fo-Fc map (contoured at 1.5 σ) around the MPD is also shown. Full size image In the crystal structures of both γ-HL-WR and LUK determined in this study, the upper and bottom halves of the β-barrel corresponding to extra- and transmembrane regions, respectively, had different structural properties, that is, a rigid β-barrel structure for the upper half and a flexible structure for the bottom half, although these two regions finally fold into a rigid single β-barrel structure. These results indicated that the extra- and transmembrane regions are formed independently. It should be noted that the intact β-barrel pore is highly stable and does not dissociate even in the presence of 1% SDS [20] , [21] , [25] , [26] , [27] . It was surprising that such a stable structure was composed of two parts that form independently. γ-HL-WR was reported to form a ring-shaped oligomer on the erythrocyte surface but to have no haemolytic activity. Moreover, the oligomer of γ-HL-WR was sensitive to 1% SDS [10] . LUK also formed a ring-shaped oligomer on the human erythrocyte surface, although it did not show haemolytic activity towards human erythrocyte ( Fig. 3b and Supplementary Fig 3 ). The determined oligomeric structures with a highly flexible bottom half of the β-barrel reasonably explain these molecular characteristics. That is, the inability to form a transmembrane β-barrel would cause SDS-sensitive inactive oligomer formation. The fluorescent spectra of pore and prepore on erythrocytes prepared using BADAN-labelled Hlg2 suggested that the prepore differs from the pore in the bottom part of the β-barrel ( Fig. 2 ). These coincidences between structural and biochemical properties indicated that the crystal structures determined in this study corresponded to the prepore state oligomer observed on erythrocytes. Crystal packing of LUK, in which the space of the transmembrane region was occupied by the adjacent octamer, demonstrated that the observed structure is definitely distinct from the pore possessing a transmembrane β-barrel ( Supplementary Fig. 4 ). In the crystallization method used, spontaneous assembly of monomers into octamers and subsequent crystallization of the octamer occurred in a crystallization drop with the aid of MPD, indicating that the observed octamer with a disordered transmembrane region must exist as a semistable state under the crystallization conditions used. On the other hand, previously reported pore structures commonly had high B-values in the transmembrane region. The flexible propensity of the region in the pore would be due to the original disordered structure of the region in the prepore state. The prepore structure model that was constructed by superposing the monomeric structure onto the octameric pore showed steric hindrance of the prestem held inside the cap domains with the adjacent protomer [21] . The crystal structures of γ-HL-WR and LUK avoided such steric hindrance, as the stem regions were not folded but extruded to form the upper half of the β-barrel ( Figs 1a and 4a ). Prepore state oligomers have been trapped previously using mutants in which disulphide linkage was artificially introduced between prestem and cap domain or within prestem [12] , [28] , [29] . Most of these oligomers were weakly assembled, and were observed only in the presence of chemical cross-linker [29] . The observed weakly assembled oligomers of the disulphide-linked mutants might be formed by exploiting the intrinsic flexibility of the prestem to avoid the steric hindrance. Since these artificial disulphide linkages are not formed in nature, much larger conformational change, as observed in the present study, could occur to form stable prepore after assembling. Taken together, we propose the following two-step β-barrel formation mechanism ( Fig. 5 steps 4–5): (i) the extramembrane region (upper half) of the β-barrel is formed coupled with oligomer formation, although the transmembrane half (bottom half) is still highly flexible in this state (prepore state); and then (ii) the flexible transmembrane region folds into a rigid β-barrel to finally form the membrane-spanning pore ( Fig. 5 ). 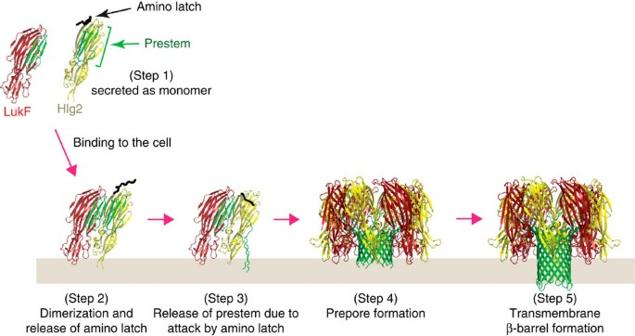Figure 5: Proposed pore formation mechanism. (Step 1): each PFT is secreted as soluble monomer. (Step 2): Hlg2 and LukF form a dimer on the cell surface. By releasing the amino latch located beside the cap domain, interprotomer interactions are formed adequately. (Step 3): the prestem extends due to attack by the released amino latch. On extension, the prestem is completely unfolded. (Step 4): dimers assemble to octameric prepore. In the prepore state, only the extramembrane half of the β-barrel is formed. (Step 5): the transmembrane half of the β-barrel is inserted into the membrane, and pore formation is completed. Figure 5: Proposed pore formation mechanism. (Step 1): each PFT is secreted as soluble monomer. (Step 2): Hlg2 and LukF form a dimer on the cell surface. By releasing the amino latch located beside the cap domain, interprotomer interactions are formed adequately. (Step 3): the prestem extends due to attack by the released amino latch. On extension, the prestem is completely unfolded. (Step 4): dimers assemble to octameric prepore. In the prepore state, only the extramembrane half of the β-barrel is formed. (Step 5): the transmembrane half of the β-barrel is inserted into the membrane, and pore formation is completed. Full size image Structure comparison of the Hlg2 protomer in γ-HL prepore with monomeric LukS-PV showed that the amino latch in the prepore occupied a region in which the prestem was located in the monomer ( Fig. 1d ). Moreover, the area in which the amino latch was located in the monomer was used for interacting with the adjacent protomer in the prepore. These observations indicated that the amino latch located beside the cap domain is released due to the approach of the adjacent protomer, and then the released amino latch interferes with the prestem, which triggers its extrusion ( Fig. 5 steps 1–3). The extruded prestems form the extramembrane region of the β-barrel by assembling to an octamer, which completes the prepore formation step ( Fig. 5 steps 3–4). Through this process, the prestem would be released in each step of assembling new protomers, and the extramembrane β-barrel would be formed by gradual addition of the stem from each protomer. It should be noted that all intramolecular hydrogen bonds within the prestem are disrupted, and new hydrogen bonds are formed within and between protomers instead. The driving force of the dramatic conformational changes on assembly would be supplied by the favourable enthalpy of these hydrogen bonds. The remaining issue to be discussed is the trigger(s) of the transmembrane pore formation. LUK (LukS and LukF) was crystallized as prepores, whereas wild-type γ-HL (Hlg2 and LukF) formed pores under similar crystallization conditions [21] . In both structures, MPD was bound at the lipid-head-binding pocket of LukF ( Fig. 4c ). These observations indicated that the influence of MPD binding on LukF is not equivalent between LUK and γ-HL. The order of binding of each component on the target cell membrane is opposite between LUK and γ-HL [30] , [31] . That is, LukF binds to the target cell first in γ-HL [30] , whereas LukS binds first in LUK [31] , suggesting that LukF plays different roles in LUK and γ-HL. LUK may not be satisfied solely with MPD binding with LukF but may require some other stimulation to form pores. A conformational change of LukS on interacting with the cell surface may be necessary. On the other hand, substitution of Trp177 and Arg198 responsible for lipid-head binding interrupts pore formation in γ-HL [10] ( Fig. 3a ), indicating a pivotal role of lipid-head binding on pore formation. Potrich et al . [32] reported that γ-HL required the freely accessible head of phosphatidylcholine to bind to the membrane. To cope with the mechanical counteraction coupling with insertion of the stem into the membrane, stable binding using Trp177 and Arg198 may be essential. The pore-forming ability was markedly influenced by the composition of the lipid membrane [32] . Trp177 and Arg198 may also be involved in disrupting the local structure of the membrane. Recently, the molecular basis underlying the biogenesis of β-barrel outer membrane proteins was reported, in which a chaperone protein (BAM) locally destabilizes the membrane to assist insertion of the outer membrane protein β-barrel into the membrane [33] . Trp177 and Arg198 may disrupt the membrane structure to facilitate insertion of the β-barrel pore into the membrane. The results of mutation analysis indicated a critical role of Gly120 of LukF in haemolytic activity ( Fig. 3a ). As Gly120 of LukF and the counterparts of S-components (hereafter these relevant glycines are represented together as Gly120s) are the first residues of the invisible transmembrane β-barrel in the prepore structure, Gly120s should act as a joint between the rigid upper half and flexible bottom half of the β-barrel. In pore structures, Gly120s are located at the middle of the β-strand and participate in the β-barrel ( Supplementary Fig. 2A ). On the other hand, in the monomer, they are located in a turn at the top of the prestem, which enables the prestem to fold in a compact conformation beside the cap domain ( Supplementary Fig. 2B ). Moreover, Gly120s in the monomer formed hydrogen bonds with Asp44 in a loop located at the top of the cap domain (hereafter loop-A following ref. 21 ) ( Supplementary Fig. 2C ). In dihedral angle analysis, Gly120s in the monomer and pore were shown to be concentrated in narrow regions in the Φ–Ψ plane ( Supplementary Fig. 5A ), indicating that Gly120s have certain rigid conformations in both monomer and pore, whereas they are flexible in the prepore. Gly120s should have to change the conformation from a rigid turn structure to a rigid β-barrel via the flexible state. The rigid conformation in the monomer may be necessary to fasten the prestem with loop-A ( Supplementary Fig. 2B,C ). To enable such a conformational change, the residue at this position would have to be glycine. Taken together, Gly120s are likely to have two important roles, that is, (i) acting as a joint to fold the long stem into the compact prestem, and (ii) acting as a clasp to fasten the prestem with loop-A. It is reasonable to use a single residue for these two distinct purposes. In contrast to Gly120, substitution of Gly135 increased haemolytic activity ( Fig. 3a ). Gly135 was located at the interface between extra- and transmembrane parts of the β-strand coming back to the rim domain ( Supplementary Fig. 2A ). This residue was disordered in five of seven monomer structures reported previously [13] , [14] , [15] , [16] , [17] . Even in two structures in which Gly135s have been traced, they were dispersed in the Φ-Ψ plane ( Supplementary Fig. 5B ). These observations suggest that Gly135s do not have a static conformation and can adopt any conformation freely in the monomer. Substitution of Gly135 may cause fixing of a conformation preferable for pore formation, which would result in activation. Substitution of other glycines in the transmembrane region caused moderate inactivation ( Fig. 3a ). In the monomer, a large part of the transmembrane region was disordered ( Supplementary Fig. 2B ). Each Gly alone would contribute to the intrinsic flexibility of the region. Incomplete inactivation by substitution for Pro would be due to its intrinsic property of flexibility ranging over this region, that is, conformational fixation at one residue was cancelled by the highly flexible propensity. In the prepore state, the transmembrane regions from eight protomers are expected to gather in a narrow space within the upper half of the β-barrel. Glycine possessing the smallest side chain may reduce bulk in addition to its flexible properties. With the determination of the prepore state structure in this study, all structures of the monomer, prepore and pore of γ-HL have become available. The two-step β-barrel formation mechanism proposed based on these structures clearly explains the pore formation process with no stereochemical discrepancies. As the flexibility of the transmembrane part was observed in both γ-HL-WR and LUK, we conclude that the mechanism is adopted by all staphylococcal two-component PFTs regardless of the kind of components. Moreover, based on the results of biochemical analysis, Sato et al . [34] recently showed that the transmembrane β-hairpin of perfringolysin O, a bacterial cholesterol-dependent cytolysin, was unfolded and had freedom of motion in the prepore state, which agreed with the present structural data, although the molecular architecture of perfringolysin O is entirely different from those of staphylococcal β-PFTs. On the other hand, the pore formation mechanism recently proposed for aerolysin based on the cryo-electron miccroscopy structures—a swirling membrane insertion mechanism—is fundamentally different [35] . There should be diversity in the mode of action although the β-barrel architecture is commonly used as a transmembrane pore. It is significant to determine the molecular mechanisms of action of other superfamilies and discuss differences and similarities. Crystal structure analysis LukF, Hlg2, LukS and their mutants were overexpressed with His6-tags at their N-termini in Escherichia coli , and purified as soluble monomeric proteins using His Trap and HiLoad 26/60 Superdex 200-pg columns (GE Healthcare). The 1:1 mixtures of W177A/R198A mutant of LukF and Hlg2 or wild-type LukF and LukS were concentrated to 10 mg ml −1 , and then used for crystallization. Crystallization was performed by the sitting-drop vapour diffusion method at 293 K. The crystals of γ-HL-WR were grown from a buffer containing 60% MPD, sodium acetate (pH 4.8) and 0.15 M disodium hydrogen phosphate. Crystals of LUK were grown from a buffer composed of 40% MPD, sodium acetate (pH 4.8) and 0.15 M disodium hydrogen phosphate. X-ray diffraction experiments were performed at Photon Factory (Tsukuba, Japan) and SPring-8 (Harima, Japan) under proposals 2012G515/2014G022 and 2012A1179, respectively. X-ray diffraction data sets of γ-HL-WR and LUK were collected on the beamline BL1A at Photon Factory and BL41XU at SPring-8, respectively. The diffraction data were indexed, integrated, scaled and merged using the programs XDS and XSCALE [36] . The data statistics are shown in Table 1 . Crystal structures were determined by the molecular replacement method with the programme Phaser [37] . The structure of γ-HL (PDB 3B07) of which the stem regions were truncated was used as a search probe. To monitor the refinement, a random 5% subset of γ-HL and 1% subset of LUK were set aside for calculation of the R free factor. After rigid body refinement and manual model building with Coot [38] , and individual atomic coordinate refinement and individual ADP refinement were performed with individual atomic coordinates using phenix.refine [39] . The refinement statistics are summarized in Table 1 . Table 1 Data collection and refinement statistics. Full size table Haemolysis assay Aliquots of 1 ml of 5% human or rabbit erythrocytes were incubated with 0.6 μg of each purified component protein at 37 °C for 30 min, followed by centrifugation at 2,000 g for 30 min at 10 °C. The supernatant was diluted 10-fold with tris-buffered saline buffer, and then the absorbance of released haemoglobin at 540 nm was measured using a DU800 spectrophotometer (Beckman Coulter). Analysis of emission profile of BADAN Each cysteine-substituted Hlg2 was incubated with 10 mM BADAN for 2 h at room temperature, followed by removal of the unreacted molecules using Vivaspin 500 ultrafilter (GE Healthcare). Procedures of emission shift analysis of BADAN-labelled Hlg2 mutants in the pore or prepore were, in principle, those followed by Nguyen et al . [9] Briefly, BADAN-labelled Hlg2 cysteine mutants (1.6 μg) and equal amounts of LukF or LukF W177A/R198A mutant were incubated with right-side-out resealed-membrane ghosts prepared from 50 μl of 50% human erythrocytes at 37 °C for 30 min in PBS. After centrifugation at 5,000 g for 5 min at 4 °C, the precipitant was washed and resuspended by PBS. The fluorescence of BADAN-labelled proteins was measured using F-2500 fluorescence spectrophotometer (Hitachi) (lambda ex=408 nm, 5-nm bandpass; lambda em=440–600 nm, 5-nm bandpass). How to cite this article : Yamashita, D. Molecular basis of transmembrane beta-barrel formation of staphylococcal pore-forming toxins. Nat. Commun . 5:4897 doi: 10.1038/5897 (2014). Accession codes : The atomic coordinates of γ-HL-WR and LUK have been deposited in the Protein Data Bank (PDB 4P1Y and 4P1X , respectively).